Two-barrier stability that allows low-power operation in current-induced domain-wall motion Energy barriers in magnetization reversal dynamics have long been of interest because the barrier height determines the thermal stability of devices as well as the threshold force triggering their dynamics. Especially in memory and logic applications, there is a dilemma between the thermal stability of bit data and the operation power of devices, because larger energy barriers for higher thermal stability inevitably lead to larger magnetic fields (or currents) for operation. Here we show that this is not the case for current-induced magnetic domain-wall motion induced by adiabatic spin-transfer torque. By quantifying domain-wall depinning energy barriers by magnetic field and current, we find that there exist two different pinning barriers, extrinsic and intrinsic energy barriers, which govern the thermal stability and threshold current, respectively. This unique two-barrier system allows low-power operation with high thermal stability, which is impossible in conventional single-barrier systems. Energy barriers often appear in diverse systems in nature and determine their dynamical, statistical and/or thermal properties [1] , [2] , [3] , [4] , [5] , [6] , [7] , [8] , [9] , [10] , [11] , [12] , [13] , [14] . For magnetization reversal dynamics, such as magnetization switching in nanomagnets [4] , [5] , [6] , [7] , [8] , [9] , [10] , [11] and magnetic domain-wall (DW) motion along nanowires [12] , [13] , [14] , [15] , [16] , [17] , the energy barrier has long been studied and is still a debatable issue, because it determines the fundamental device properties such as thermal stability and the threshold force for triggering dynamics [5] , [6] . Thus, we need to identify the energy barrier for the magnetization reversal in nanoscale devices if we are to use that reversal process in magnetic memories [18] , [19] and logics [20] . In general, there is a severe dilemma between the thermal stability of bit data and the operation power of devices, because larger energy barriers for higher thermal stability inevitably lead to larger magnetic fields (or currents) for operation. This is mainly due to a single energy barrier governing the total system dynamics. Here, we show that this is not the case for the current-induced magnetic DW motion induced by the adiabatic spin-transfer torque. We investigated DW depinning from a well-defined site in a ferromagnetic Co/Ni nanowire, and found that the depinning barrier for the field-induced motion is much larger than that for the current-induced motion. This discrepancy shows that the system has two different pinning barriers for magnetic field and electric current, which are found to be extrinsic and intrinsic energy barriers, respectively. The present system is unique in that a single system has two kinds of energy barriers, which govern the thermal stability and threshold current, respectively. This peculiar nature originating from the internal degree of freedom of a DW is technologically useful, because it allows the low-power operation with high thermal stability through independent tune of these barriers, which is impossible in a single-barrier system such as the conventional magnetic storage devices. Device structure and measurement procedure A scanning electron microscope image of our device structure and a schematic illustration of our measurement setup are shown in Fig. 1a . Several nanowires ( w =80–90 nm, L =6 μm) designed with Hall cross structure were patterned by electron-beam lithography and ion milling from a Si/Ta(3 nm)/Pt(1.5 nm)/Co(0.3 nm)/[Ni(0.9 nm)/Co(0.3 nm)] 4 /Pt(1.5 nm)/Ta(3 nm) film. Two Ti(5 nm)/Au(100 nm) electrodes (labeled A and B in the figure) were attached to inject current to nucleate and push the DW. The Hall cross structure connected to Ta electrodes was designed to pin the DW and detect the DW depinning by means of the anomalous Hall effect (AHE). A direct current of 20 μA (corresponding current density flowing along the Co/Ni layer is ~2.5 × 10 10 A m −2 ) was used for AHE resistance measurement. All the measurements were performed at room temperature (300±1 K). 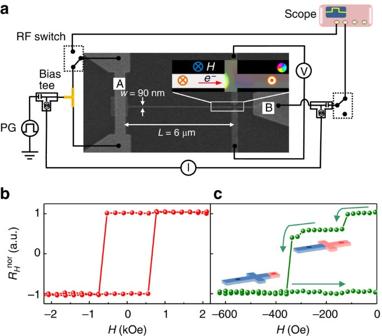Figure 1: Device structure with measurement setup and Hall measurement for DW initialization. (a) Scanning electron microscope image of the device is combined with a schematic drawing of the measurement setup. The high-magnification inset shows a snapshot (obtained by micromagnetic simulation) of the pinned DW at the Hall cross. Color represents the internal magnetization direction. PG, pulse generator. (b) Result of the AHE measurement of the wire. The vertical axis is normalized AHE resistance (1 for upward magnetization and −1 for downward). (c) Normalized AHE resistance measured after initializing the DW by sweeping the magnetic field toward the negative direction. The snapshot images denote the magnetization configurations of the low-field (|H1|<|H|<|H2|) and high-field (|H|>|H2|) regions. Figure 1: Device structure with measurement setup and Hall measurement for DW initialization. ( a ) Scanning electron microscope image of the device is combined with a schematic drawing of the measurement setup. The high-magnification inset shows a snapshot (obtained by micromagnetic simulation) of the pinned DW at the Hall cross. Color represents the internal magnetization direction. PG, pulse generator. ( b ) Result of the AHE measurement of the wire. The vertical axis is normalized AHE resistance (1 for upward magnetization and −1 for downward). ( c ) Normalized AHE resistance measured after initializing the DW by sweeping the magnetic field toward the negative direction. The snapshot images denote the magnetization configurations of the low-field (| H 1 |<| H |<| H 2 |) and high-field (| H |>| H 2 |) regions. Full size image Figure 1b shows the AHE resistance measured while sweeping an external magnetic field along the perpendicular direction. The AHE resistance was normalized to its saturation value: =1 when the direction of magnetization at the Hall cross is upward, and −1 when it is downward. Clear square hysteresis is observed, indicating the perpendicular magnetic easy axis of the nanowire. In order to initialize a DW at the Hall cross, we first saturated the nanowire to the upward direction by applying sufficiently large magnetic field of 2 kOe. The pulse generator (PG in Fig. 1a ) then injected a pulse current (−60 mA, 15 ns) into electrode A to nucleate the DW by generating a local Oersted field. Subsequently, we swept the magnetic field to the downward direction to push the DW to the Hall cross. As the magnetic field strength increased, we observed two steps of ( Fig. 1c ). The first (at H 1 =−150 Oe) corresponds to the DW arrival at the left part of Hall cross, and the second (at H 2 =−350 Oe) corresponds to the depinning from the Hall cross [21] , [22] . To initialize the DW at Hall cross, we applied H =−250 Oe after DW nucleation and then returned H to 0 Oe. In all the measurements, we confirmed by measuring that the DW was repeatedly positioned at the Hall cross. Determination of energy barrier for magnetic field First, we determined the energy barrier for DW pinning due to the geometrical constriction of Hall bar structure by using a magnetic field as the driving force for depinning the DW. This is the conventional method for estimating the thermal stability of the magnetic device. We first initialized the DW at the Hall cross as described above and then applied a magnetic field while monitoring . At a certain time, the depinning time t d , dropped abruptly ( Fig. 2a ), indicating the depinning of DW from the Hall cross. We have confirmed by repeated measurement that signal drop does not involve a stair-like behavior, which means that there are no additional pinning sites in the Hall cross ( Fig. 2a ). The depinning is thus due to the overcoming of a single energy barrier. 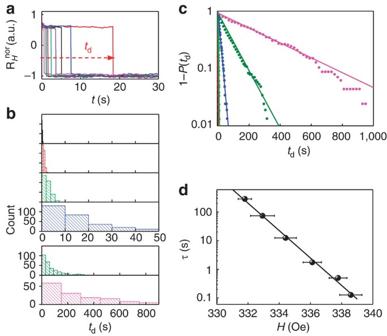Figure 2: Quantitative determination of extrinsic energy barrier. (a) Typical examples of time evolution of AHE signal for magnetic-field-driven DW depinning. (b) Distributions of depinning timetdat various magnetic field strengths: 338.6 Oe (black), 337.8 Oe (red), 336.1 Oe (green), 334.4 Oe (blue), 332.9 Oe (olive) and 331.8 Oe (magenta). Histograms were obtained from 300 repeated measurements except for 331.8 Oe (100 measurements). (c) Cumulative distribution function oftdvalues whose histograms are shown inFig. 2b. Different colors correspond to the different field strengths, which is same withFig. 2b. Solid lines are the best-fit lines based on the equationP(td)=1−exp(−td/τ). (d) Characteristic depinning timeτas a function of magnetic field obtained fromFig. 2c. Error bars show s.d., and the solid line is the best-fit line based on the Arrhenius law. Figure 2b shows histograms of the depinning time t d obtained from 300 repeated measurements at various magnetic field strengths. To determine the energy barrier in the thermally activated regime ( H << H th ), we examined depinning times ranging from 0.1 s to 1,000 s. Cumulative distribution function for each magnetic field is presented in Fig. 2c , which is well fitted by simple exponential function with a single characteristic depinning time τ : P ( t d )=1−exp(− t d / τ ). Clear exponential decay with a single τ shows that this process is indeed governed by a single energy barrier. We note that the single energy barrier is not the case in wide wires (see Supplementary Fig. S1 and Supplementary Note 1 ). Figure 2: Quantitative determination of extrinsic energy barrier. ( a ) Typical examples of time evolution of AHE signal for magnetic-field-driven DW depinning. ( b ) Distributions of depinning time t d at various magnetic field strengths: 338.6 Oe (black), 337.8 Oe (red), 336.1 Oe (green), 334.4 Oe (blue), 332.9 Oe (olive) and 331.8 Oe (magenta). Histograms were obtained from 300 repeated measurements except for 331.8 Oe (100 measurements). ( c ) Cumulative distribution function of t d values whose histograms are shown in Fig. 2b . Different colors correspond to the different field strengths, which is same with Fig. 2b . Solid lines are the best-fit lines based on the equation P ( t d )=1−exp(− t d / τ ). ( d ) Characteristic depinning time τ as a function of magnetic field obtained from Fig. 2c . Error bars show s.d., and the solid line is the best-fit line based on the Arrhenius law. Full size image To determine the energy barrier quantitatively, we plotted the characteristic depinning time τ as a function of magnetic field H as shown in Fig. 2d . It is known that thermally activated DW depinning driven by magnetic field is described by τ = τ 0 exp(Δ mag / k B T ), where the energy barrier Δ mag is given by with threshold magnetic field H th . Here, the value of the exponent α depends on the reversal mechanism and is known to be α =2 for nucleation-dominant magnetization reversal and α =1 for wall-motion-dominant expansion [23] . In this work, we used α =1 because the wall motion is dominant in our device [24] . We have confirmed that the backward-hopping rate is negligible in our device due to the high depinning magnetic field [25] . An exponential fit (solid line in Fig. 2d ) gives 16.2±0.5 × 10 −19 J (corresponds to 392±13 k B T for T =300 K) for the energy barrier Δ mag,0 , by assuming an attempt frequency of =1 GHz. Here, we note that the imprecision of τ 0 does not substantially affect the estimation of the energy barrier, as the reported values [6] , [7] , [8] , [9] , [10] , [11] , [12] , [13] , [14] , [15] , [16] , [26] of τ 0 from 24 ps to 1 ns gives an energy barrier correction term of |4 k B T |, which is less than the experimental error. Determination of energy barrier for electric current Next, we determined the energy barrier by using an electric current as the driving force for depinning the DW. After initializing the DW at the Hall cross, a direct current was applied from electrode B to A while monitoring . At a certain time, the depinning time t d , dropped abruptly ( Fig. 3a ), indicating DW depinning from the Hall cross. To perform statistical analysis, we repeated this procedure 300 times for each current strength. Histograms of t d at several current strengths are shown in Fig. 3b . The cumulative distribution function for each current ( Fig. 3c ) is also presented, which is well fitted by a simple exponential function with a single characteristic depinning time τ . Clear exponential decay with a single τ manifests that the current-induced DW depinning is governed by a single energy barrier. 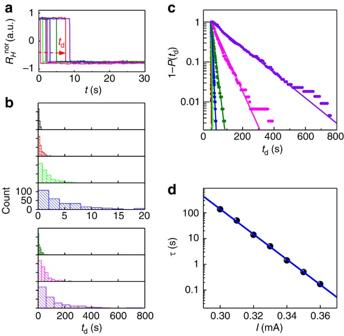Figure 3: Quantitative determination of intrinsic energy barrier. (a) Typical examples of time evolution of AHE signal for electric-current-driven DW depinning. (b) Distributions of depinning timetdat various current strengths: 0.36 mA (black), 0.35 mA (red), 0.34 mA (green), 0.33 mA (blue), 0.32 mA (olive), 0.31 mA (magenta) and 0.30 mA (purple). All histograms were obtained from 300 repeated measurements. Here, the current is the value flowing along the magnetic layer (Co/Ni) (c), Cumulative distribution functions of thetdvalues whose histograms are shown inFig. 3b. Different colors correspond to the different current strengths, which is same withFig. 3b. Solid lines show the best fittings to the formP(td)=1−exp(−td/τ). (d) Characteristic depinning timeτas a function of current obtained fromFig. 3c. Error bars show s.d., and the blue solid line is the best-fit line based on the Arrhenius law. Figure 3: Quantitative determination of intrinsic energy barrier. ( a ) Typical examples of time evolution of AHE signal for electric-current-driven DW depinning. ( b ) Distributions of depinning time t d at various current strengths: 0.36 mA (black), 0.35 mA (red), 0.34 mA (green), 0.33 mA (blue), 0.32 mA (olive), 0.31 mA (magenta) and 0.30 mA (purple). All histograms were obtained from 300 repeated measurements. Here, the current is the value flowing along the magnetic layer (Co/Ni) ( c ), Cumulative distribution functions of the t d values whose histograms are shown in Fig. 3b . Different colors correspond to the different current strengths, which is same with Fig. 3b . Solid lines show the best fittings to the form P ( t d )=1−exp(− t d / τ ). ( d ) Characteristic depinning time τ as a function of current obtained from Fig. 3c . Error bars show s.d., and the blue solid line is the best-fit line based on the Arrhenius law. Full size image As shown in Fig. 3d , τ is found to depend on the current exponentially, which reflects the thermally assisted DW depinning. In this thermally activated regime, theory [27] predicts that τ should follow the Arrhenius-law-based exponential equation τ = τ 0 exp(Δ cur / k B T ), where Δ cur = with effective threshold current, . The exponential fit (blue solid line in Fig. 3d ) gives the energy barrier of =2.5±0.1 × 10 −19 J (corresponds to 60±3 k B T for T =300 K), by assuming an attempt frequency of =1 GHz. Surprisingly, the energy barrier obtained by using an electric current as the driving force is much smaller than that determined by using a magnetic field. To check the validity of the barrier obtained by using the current, we examined the barrier in other regimes of DW dynamics, that is, the flow regime, by injecting higher current through the wire. We used pulse currents with fixed duration t p and measured depinning probability at various current strengths. We first initialized the DW at the Hall cross and monitored before and after injecting the current pulse to check the depinning of DW. Depinning probability was calculated from the results of 10 measurements at each current strength and duration. In Fig. 4a , the total DW depinning probability ( P ) is plotted against current and current density. Note that the P -versus- I distributions for short pulse durations ( t p <100 ns) are wider than those for long pulse durations ( t p =1 μs–0.1 s), which implies different dynamic regimes of DW depinning (flow regime and thermally activated regime). 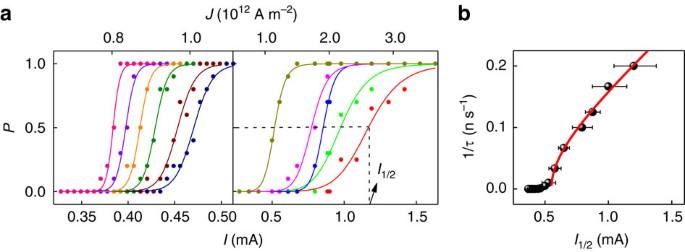Figure 4: Quantitative determination of intrinsic energy barrier for flow regime. (a) Depinning probability as a function of current (lower abscissa) and current density (upper abscissa) for various pulse durationstp: 5 ns (red), 6 ns (green), 8 ns (blue), 10 ns (magenta), 100 ns (dark yellow), 1 μs (navy), 10 μs (wine), 100 μs (olive), 1 ms (orange), 10 ms (violet) and 100 ms (pink). Each data point was determined from 10 measurements. Solid lines are the probability fitting curves. (b) 1/τas a function of currentI1/2. TheτandI1/2are respectively the pulse duration and current that giveP=1/2. The error bars correspond to 20/80% probabilities, and the red solid line is the fitting to, withAbeing a prefactor. Figure 4: Quantitative determination of intrinsic energy barrier for flow regime. ( a ) Depinning probability as a function of current (lower abscissa) and current density (upper abscissa) for various pulse durations t p : 5 ns (red), 6 ns (green), 8 ns (blue), 10 ns (magenta), 100 ns (dark yellow), 1 μs (navy), 10 μs (wine), 100 μs (olive), 1 ms (orange), 10 ms (violet) and 100 ms (pink). Each data point was determined from 10 measurements. Solid lines are the probability fitting curves. ( b ) 1/ τ as a function of current I 1/2 . The τ and I 1/2 are respectively the pulse duration and current that give P =1/2. The error bars correspond to 20/80% probabilities, and the red solid line is the fitting to , with A being a prefactor. Full size image To clarify the flow regime, we plotted 1/ τ against current as shown in Fig. 4b . Here, τ and I 1/2 were defined as the pulse duration and the current when P =1/2, respectively. It is clear that there is a threshold current I th , which was predicted by a theory based on the adiabatic STT model [28] , [29] . In this model, the energy barrier that can be described by =2 ΩλK d (where Ω is the cross-sectional area, λ is the DW width parameter and K d is the effective DW anisotropy) gives rise to the threshold current density to move the DW. This threshold current density, J th , is calculated by J th =( eγλ / pμ B ) K d , where e is the charge carried by a single electron, γ is a gyromagnetic ratio, p is spin polarization and μ B is the Bohr magneton. Thus, one can easily obtain the energy barrier by determining the threshold current I th , as =2 pμ B I th / eγ . The energy barrier in our device is determined, from the threshold current of I th =0.55±0.01 mA (red fitting line in Fig. 4b ), to be =2.4±0.2 × 10 −19 J (corresponds to 59±6 k B T for T =300 K). Here, we used P =0.66±0.06, which was determined in a previous experiment [30] . The two energy barriers obtained by analyses of different dynamic regimes (flow regime and thermally activated regime) are found to be consistent with each other, indicating the validity of the determination of the energy barrier. Thus, it was confirmed that there is a huge discrepancy between the energy barriers determined by using magnetic field and electric current. This discrepancy can be successfully resolved if we accept the idea that the system has two different pinning barriers depending on whether it is driven by the magnetic field or the electric current. Two barriers for magnetic DW motion For a DW motion along the nanowire ( Fig. 5a ), it is known that there are two different energy barriers, one extrinsic and the other intrinsic [28] , [31] . Figures 5b and c show schematic energy landscapes of a DW, with and without d.c. current, respectively, as functions of two collective coordinates q and φ defined in Fig. 5a . The extrinsic energy barrier is due to geometrical artefacts such as inevitable edge/surface roughness and defects or intentionally formed notch structures [14] , [15] , [16] , [32] , [33] , [34] . Thus, the distribution of extrinsic energy barrier usually shows large fluctuation depending on the position q and consequently, the DW motion exhibits extremely stochastic behavior, as observed in field-driven DW motion [34] . The intrinsic energy barrier, on the other hand, is defined by internal energy difference between Bloch and Néel walls and is not affected by geometrical artefacts. A recent experiment has shown that intrinsic pinning determines the threshold for current-induced DW motion due to adiabatic spin-transfer torque [17] . Thus, one can conclude that the two different energy barriers obtained by magnetic field and current correspond to the extrinsic and intrinsic energy barrier, respectively. 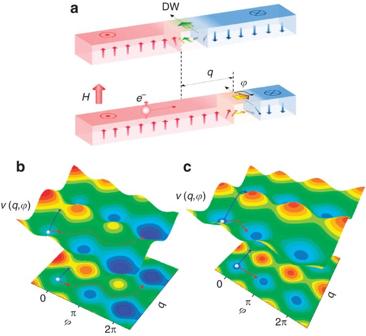Figure 5: Schematic illustration of DW motion and energy landscape. (a) A magnetic DW in a nanowire and its collective coordinates, the positionqand the tilting angleφ. (b,c), Energy landscape for the DW motion in the presence (b) and absence (c) of d.c. current. Here, the periodic potential alongqdirection is not the exact energy barrier but an illustrative one to represent typical energy barrier. In (b), the d.c. current tilts the potential in theφdirection. Once the DW is excited above the intrinsic barrier (indicated by the red solid arrow), it evolves dynamically along the red dotted curve and eventually overcomes the extrinsic barrier, which is lowered by the tilting. Note that the threshold is determined by the intrinsic barrier when the intrinsic barrier is lower than the extrinsic one. Thermal excitation overcoming the extrinsic pinning potential alongqaxis (blue arrow) is blocked due to high-energy barrier. In (c), there is no tilting in the energy landscape. When the intrinsic barrier is lower than the extrinsic one, the DW may easily overcome the intrinsic barrier (red arrow), but this does not lead to the depinning from the extrinsic barrier since it does not changeq. The DW depinning from the extrinsic pinning occurs only when it overcomes the full extrinsic barrier (blue arrow). Figure 5: Schematic illustration of DW motion and energy landscape. ( a ) A magnetic DW in a nanowire and its collective coordinates, the position q and the tilting angle φ . ( b , c ), Energy landscape for the DW motion in the presence ( b ) and absence ( c ) of d.c. current. Here, the periodic potential along q direction is not the exact energy barrier but an illustrative one to represent typical energy barrier. In ( b ), the d.c. current tilts the potential in the φ direction. Once the DW is excited above the intrinsic barrier (indicated by the red solid arrow), it evolves dynamically along the red dotted curve and eventually overcomes the extrinsic barrier, which is lowered by the tilting. Note that the threshold is determined by the intrinsic barrier when the intrinsic barrier is lower than the extrinsic one. Thermal excitation overcoming the extrinsic pinning potential along q axis (blue arrow) is blocked due to high-energy barrier. In ( c ), there is no tilting in the energy landscape. When the intrinsic barrier is lower than the extrinsic one, the DW may easily overcome the intrinsic barrier (red arrow), but this does not lead to the depinning from the extrinsic barrier since it does not change q . The DW depinning from the extrinsic pinning occurs only when it overcomes the full extrinsic barrier (blue arrow). Full size image Effect of Joule heating The estimation of an energy barrier, particularly in the thermally activated regime, might be affected by the device temperature, which could be increased by Joule heating. To estimate the possible effect of Joule heating on the determination of energy barrier, we obtained the device temperature by measuring temperature-dependent device resistance. Recording the current pulse in a serially connected oscilloscope allowed us to estimate the device temperature as well as the temperature rising time [35] , which is found to be below 2 ns. 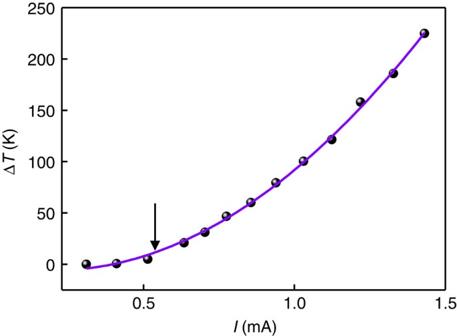Figure 6: Estimation of Joule heating. Device temperature increase as a function of currentImeasured by temperature-dependent device resistance. Arrow denotes the threshold currentIthfor DW depinning. Purple solid line is the fitting curve of Joule heating. Figure 6 shows the device temperature increase (Δ T ) as a function of current I , which was obtained by 10-ns current pulse. The temperature increase is seen to be negligible (at most +3 K) at low current ( I << I th ) and to increase gradually with increasing current, reaching 250 K at I =1.5 mA. We estimated the possible error of characteristic depinning time τ arising from Joule heating in thermally activated regime. The maximum error τ err with the temperature variation of +3 K is found to be ~20% of τ , which is comparable to the statistical error. As the variation of τ due to current is substantial (three orders of magnitude) in our experiment, such a small temperature variation does not affect the determination of the energy barrier in thermally activated regime ( I << I th ). Figure 6: Estimation of Joule heating. Device temperature increase as a function of current I measured by temperature-dependent device resistance. Arrow denotes the threshold current I th for DW depinning. Purple solid line is the fitting curve of Joule heating. Full size image We also investigated the robustness of the energy barrier determined by the threshold current I th in a short time scale. In the one-dimensional model, the intrinsic energy barrier does not depend on material parameters such as saturation magnetization ( M S ) and anisotropy ( K U ), but depends only on the threshold current I th and spin polarization p . As shown in Fig. 4b (compared with Fig. 6 ), the determination of I th is straightforward and the variation of p is negligible at I th , which was proved in our recent work [30] . Therefore, the rise in temperature by Joule heating does not affect the determination of energy barrier in the flow regime. The existence of two different energy barriers for DW motion is advantageous for application: reducing the threshold current density while maintaining the thermal stability. It is because the intrinsic energy barrier is irrelevant to the thermal stability, though it determines the threshold current. To understand it, it is important to realize a crucial difference between the cases with and without d.c. current. In the presence of d.c. current, the energy landscape is tilted in the φ direction (see Fig. 5b ). Once a DW gets over the intrinsic barrier, it moves downstream in the φ direction, and finds a point where the extrinsic barrier is sufficiently lowered and can be overcome. This process is indicated by the red arrow in Fig. 5b . This explains why the intrinsic barrier determines the threshold for the DW depinning from the extrinsic barrier. On the other hand, the thermal stability for practical use is properly determined in the absence of d.c. current. Therefore, for a DW to move in the q direction, it must overcome the full extrinsic barrier as there is no lowering due to current (no tilt in the energy landscape). This process is indicated by the blue arrow in Fig. 5c . As a possible exception, a sufficiently large current may arise spontaneously (as a fluctuation in the equilibrium) and induce the depinning process. Some analysis, however, shows that the probability for this is extremely small (see Supplementary Fig. S2 and Supplementary Notes 2 and 3 ). Therefore, it is concluded that thermal stability is determined solely by the extrinsic barrier, and the intrinsic barrier is irrelevant; even if the intrinsic barrier is much lower than the extrinsic barrier and, thus, the DW can easily overcome the intrinsic barrier (red arrow in Fig. 5c ), it does not damage the thermal stability as far as the position of the DW is concerned. On the other hand, the threshold for the DW manipulation by current (depinning from the extrinsic pinning) is determined by intrinsic pinning. This argument can hold for the intermediate pinning regime, where the intrinsic energy barrier is independent from the extrinsic energy barrier. To identify the pinning regime, we tested the variation of energy barriers from several devices (D1, D2 and D3) that had similar wire widths (80–90 nm). The results are summarized in Fig. 7 . It is clear from the figure that intrinsic energy barriers are insensitive to the wide variation of extrinsic energy barriers, indicating that our devices belong to the intermediate pinning regime. 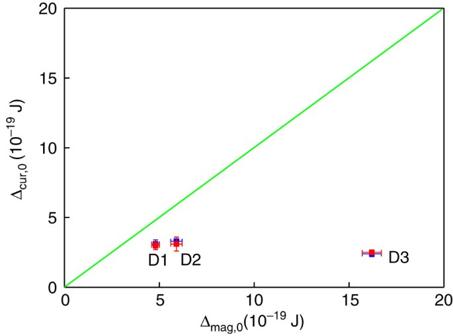Figure 7: Variation of energy barriers. Total energy barriers obtained from three different devices D1, D2 and D3. Intrinsic energy barrier Δcuris plotted with respect to the extrinsic energy barrier Δmag. Blue and red symbols corresponds toand, respectively. Green solid line denotes=. Figure 7: Variation of energy barriers. Total energy barriers obtained from three different devices D1, D2 and D3. Intrinsic energy barrier Δ cur is plotted with respect to the extrinsic energy barrier Δ mag . Blue and red symbols corresponds to and , respectively. Green solid line denotes = . Full size image In conclusion, we have experimentally demonstrated that there exist two types of energy barriers, intrinsic and extrinsic, for the DW motion, and determined both barriers quantitatively. Given that the two energy barriers can be tuned independently by proper designing of the devices [14] , [15] , [17] , this work suggests the possibility of durable spintronic devices with low power consumption. Co/Ni film preparation and device fabrication Multilayered Ta(3 nm)/Pt(1.5 nm)/Co(0.3 nm)/[Ni(0.9 nm)/Co(0.3 nm)] 4 /Pt(1.5 nm)/Ta (3 nm) film with perpendicular magnetic anisotropy was deposited on undoped Si substrates by DC magnetron sputtering. The saturation magnetization and the uniaxial anisotropy constant were determined to be 6.8 × 10 5 A m −1 and 3.8 × 10 5 J m −3 . Nanowires with widths of 80–90 nm and a length of 6 μm were fabricated together with 80-nm-wide Hall cross structures. Waveguide geometry was used to inject nanosecond current pulses without distortion. Measurement Transport measurement was used to investigate the DW depinning. A pulse generator (Picosecond 10,300B, +50/−45 V with rising time<0.3 ns) was used to nucleate the DW and depin the DW from the Hall cross in a short-pulse regime (5–100 ns). A function generator (Tabor Electronics 8511, 50 MHz) was used to depin the DW in a range of 20 ns–0.1 s. A DC source was used to measure the DW depinning time greater than 0.1 s. A DC source (Yokogawa 7651, max: 30 V, 100 mA) and nanovoltmeter (Keithley 2182) were used to detect the AHE resistance. Current strength was calculated from the voltage measured in a serially connected real-time oscilloscope (DPO 7354). Non-magnetic GSG probes were used for electrical measurements. How to cite this article: Kim, K-J. et al. Two-barrier stability that allows low-power operation in current-induced domain-wall motion. Nat. Commun. 4:2011 doi: 10.1038/ncomms3011 (2013).